Evidence for distinct human auditory cortex regions for sound location versus identity processing Neurophysiological animal models suggest that anterior auditory cortex (AC) areas process sound identity information, whereas posterior ACs specialize in sound location processing. In humans, inconsistent neuroimaging results and insufficient causal evidence have challenged the existence of such parallel AC organization. Here we transiently inhibit bilateral anterior or posterior AC areas using MRI-guided paired-pulse transcranial magnetic stimulation (TMS) while subjects listen to Reference/Probe sound pairs and perform either sound location or identity discrimination tasks. The targeting of TMS pulses, delivered 55–145 ms after Probes, is confirmed with individual-level cortical electric-field estimates. Our data show that TMS to posterior AC regions delays reaction times (RT) significantly more during sound location than identity discrimination, whereas TMS to anterior AC regions delays RTs significantly more during sound identity than location discrimination. This double dissociation provides direct causal support for parallel processing of sound identity features in anterior AC and sound location in posterior AC. A number of studies support the theory that sound identity information is processed in anterior and spatial features in posterior aspects of non-primary auditory cortices (ACs) [1] , [2] , [3] , [4] , which project to distinct inferior frontal ‘what’ and posterior parietal/superior prefrontal ‘where’ areas [5] , [6] , [7] , [8] , [9] , [10] , respectively. In humans, posterior AC regions, encompassing the planum temporale (PT) and posterior superior temporal gyrus (STG), are activated by a range of audiospatial cues [3] , [11] , [12] , [13] , [14] , whereas AC areas anterolateral to Heschl’s gyrus, extending to the anterior STG and the planum polare, are sensitive to a various sound identity features [3] , [10] , [15] , [16] , [17] , [18] , [19] , [20] . Yet, several neuroimaging studies suggest that the posterior non-primary ACs also respond to non-spatial sounds, such as ‘spectral motion’ [21] and/or phonetic features [22] , [23] , which has led to an alternative interpretation that the model of separate sound identification versus localization regions in human ACs is inaccurate (see, for example, refs 22 , 24 , 25 ). However, when interpreting the existing evidence in humans, it is noteworthy that previous studies have almost exclusively used observational neuroimaging techniques that reveal correlations, but cannot prove causality, that is, that these AC areas are required for sound identification versus localization. A powerful way to causally corroborate neuroimaging-based models is to turn the participating brain areas off one by one and observe how brain functions and behaviours change. Classically, cognitive neuropsychologists have applied this kind of approach in humans by seeking double dissociations in functional deficits between subjects with different kinds of lesions. Pioneering studies in patients with lesions extending to different aspects of the temporal cortex have provided support for the AC dual-pathway model in humans [6] , [26] , [27] . However, the specificity of this approach is limited because it is rare to find patients with lesions focused to certain part of the human AC only. For example, in one previous human lesion study on the dual-pathway model [27] , the damage extended to extra-auditory frontoparietal regions, as well as to subcortical grey and white matter in almost all studied patients. Lesion studies are, further, complicated by potential differences in premorbid abilities between subjects and compensatory changes in other brain areas related to the long-term effects of the lesion. A more accurate approach, available in animal models, is reversible inactivation of individual brain regions by cooling. A recent dual-pathway study [4] showed that local cooling of posterior versus anterior auditory fields of cat AC causes selective deficits in sound localization versus identity discrimination tasks, respectively. However, analogous confirmation in humans is still lacking. Further, although the aforementioned cooling study provided strong longitudinal evidence for the lack of long-term changes in the manipulated cat AC areas [4] , other studies using the cooling technique [28] , [29] , [30] , or alternative means of local deactivation [31] or deafferentation [32] , [33] imply that a complete deactivation of any cortical region will, within minutes [30] , result in profound changes in other areas that are connected to the manipulated region. For example, pharmacological temporary deactivation of AC leads to profound changes at the preceding subcortical stages of sound processing [34] . This raises the question whether the observed behavioural changes reflect the properties of the cooled area alone or also that of other areas. Unfortunately, there are no prior studies in any species that have investigated processing of sound identity versus location information using very transient disruption of functionality (for example, brief cortical electrical stimulation) that is less likely to induce wider spread network changes or reorganization. Instantaneous (<50 ms) and local modulations of human brain activity can be non-invasively induced using transcranial magnetic stimulation (TMS). The paired-pulse TMS (ppTMS) technique is especially powerful in this regard, as applying two TMS pulses at about 1–4 ms apart with a specific intensity ratio causes short-interval intracortical inhibition (SICI), effectively creating a relatively focal ‘functional lesion’ lasting only tens of milliseconds [35] , [36] . ppTMS therefore allows one to create short-lived functional deactivations in the human brain with high spatial and temporal accuracy, and in the context of specific behavioural paradigms, to determine the functional role of the targeted areas. This technique can be applied to healthy subjects, and the short duration of the effects allows subjects to serve as their own controls, and any compensatory functional reorganization is unlikely to occur. SICI effects emerge only when a brain area receives two TMS pulses at a specific intensity ratio, which limits them to occur locally at the TMS target area [37] . In comparison with repetitive TMS, in which the target area receives trains of pulses for a longer period of time, or cooling deactivations used in animal models, ppTMS probably results in less pronounced effects in remote areas connected to the TMS target. Further, recent advances in magnetic resonance imaging (MRI)-guided online navigation systems and focal stimulation coils allow reasonably accurate targeting, influencing spatially much smaller regions than most naturally occurring lesions. To our knowledge, there are no prior studies applying TMS to different subregions of the supratemporal AC. However, we stipulated that such an approach might be fruitful, given that TMS to sound processing areas outside the superior temporal AC has separately modulated processing of auditory object identity and spatial localization. Specifically, a recent study [38] suggested that TMS of the left inferior frontal gyrus (IFG) that is associated with the auditory ‘what’ stream [1] impairs identification of sound patterns associated with words, whereas TMS of occipital and posterior parietal cortex areas, partially overlapping with the putative auditory posterior-dorsal ‘where’ auditory stream [1] , modulates sound localization performance [39] , [40] . Recently, it was also shown that repetitive TMS to inferior parietal lobule produces selective impairments in auditory motion processing [41] . Here we utilize MRI-guided ppTMS to validate the model [1] , [2] , [3] , [4] postulating separate areas for spatial versus sound identity processing in human AC. Our results demonstrate a double dissociation that supports this parallel processing model, with ppTMS to anterior AC delaying reaction times (RTs) most prominently during sound identity discrimination and ppTMS to posterior AC delaying RTs most prominently during sound location discrimination. Cortical electric-field (E-field) estimates confirm that TMS pulses reached the intended targets in all subjects. TMS effects on sound location and identity discrimination Ten normal-hearing participants were presented with Reference/Probe sound pairs ( Fig. 1 ). In the spatial task, subjects discriminated whether Probe arrived from 5° to the left or 5° to the right relative to Reference (25° to the right). In the identity task, subjects discriminated whether the amplitude-modulation (AM) frequency of Probe was one-sixth octaves lower (35.6 Hz) or higher (44.9 Hz) than that of Reference (40 Hz). The experiment was divided into eight runs, each containing 80 trials. Fifty percent of the trials did not include TMS and therefore provided baseline RT data. For the other 50% of trials, bilateral TMS was delivered 55–145 ms after the Probes, at either the anterior or the posterior non-primary ACs. 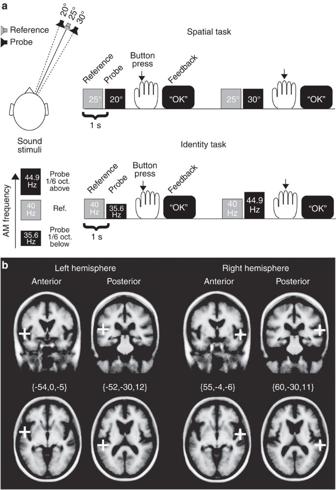Figure 1: Study design. (a) Stimuli and tasks. In the spatial task, subjects discriminated whether Probe was simulated from 5° to the left or 5° to the right relative to Reference (25° to the right). In the identity task, subjects discriminated whether Probe sound had one-sixth octaves lower or higher-AM frequency than the AM frequency of Reference (40 Hz). Feedback was presented at a computer screen after each trial in both tasks. (b) Initial TMS target locations. In 50% of the trials, paired TMS pulses were delivered 55–145 ms after Probe sound onsets, bilaterally to either the posterior or anterior AC target regions, shown here in the Freesurfer standard brain (Montreal Neurological Institute 305 or MNI305) in Talairach coordinates. For each subject, target regions were transformed through the Talairach coordinate systems. Using navigated TMS, the coil was positioned to maximally stimulate the cortical area of interest. After the experiments, TMS-induced E-fields were estimated in each subject’s cortical surface using physical modelling, to localize the maximally stimulated AC subregions (Fig. 4). Figure 1: Study design. ( a ) Stimuli and tasks. In the spatial task, subjects discriminated whether Probe was simulated from 5° to the left or 5° to the right relative to Reference (25° to the right). In the identity task, subjects discriminated whether Probe sound had one-sixth octaves lower or higher-AM frequency than the AM frequency of Reference (40 Hz). Feedback was presented at a computer screen after each trial in both tasks. ( b ) Initial TMS target locations. In 50% of the trials, paired TMS pulses were delivered 55–145 ms after Probe sound onsets, bilaterally to either the posterior or anterior AC target regions, shown here in the Freesurfer standard brain (Montreal Neurological Institute 305 or MNI305) in Talairach coordinates. For each subject, target regions were transformed through the Talairach coordinate systems. Using navigated TMS, the coil was positioned to maximally stimulate the cortical area of interest. After the experiments, TMS-induced E-fields were estimated in each subject’s cortical surface using physical modelling, to localize the maximally stimulated AC subregions ( Fig. 4 ). Full size image RT delays caused by TMS were analysed using a contemporary ‘real-time’ linear mixed modelling approach [42] , [43] (for details, see Methods) that is becoming increasingly popular amongst behavioural and cognitive scientists. This linear mixed approach models individual task responses in each task condition/subject and brings longitudinal temporal dependencies into the statistical model, thus allowing for better control for a number of biases that have been difficult to model in more traditional analyses where task responses are first aggregated within subjects [42] , [43] . For RT lags, we found task-specific modulations for the anterior versus posterior non-primary AC TMS. According to Markov chain Monte Carlo (MCMC) simulations, there was a highly significant interaction between the task-type and the TMS target location ( t =3.3, P MCMC =0.001; N Subjects =10, N Trials/Subject =640; note that conventional t / F -distributions and degrees of freedom are not directly applicable to linear mixed models). 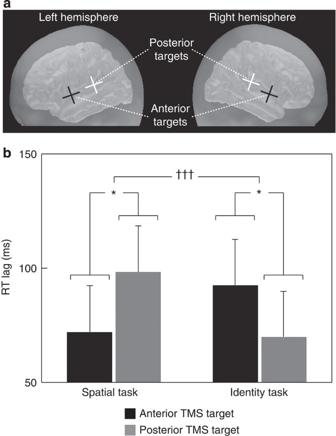Figure 2: TMS-induced RT lags during spatial and identity tasks. (a) Schematic illustration of the approximate TMS coil centre locations during bilateral anterior versus posterior stimulation. (b) Estimated marginal means and s.e. of RT lags derived from the linear mixed model, with the different stimulation latencies pooled together (N=10). These data show a significant interaction between the task and TMS target factors, suggesting brain location-specific performance modulations during auditory identity versus spatial tasks. This result provides causal support for the theory of two distinct AC areas for sound identity and location processing1,2, which has previously been suggested in humans based on neuroimaging activation studies. *P<0.05,a prioricomparison of task-specific effects across the TMS target loci derived from the linear mixed model;†††PMCMC=0.001, task by target location interaction of the linear mixed model. Figure 2 shows the estimated marginal means of RT lags caused by TMS in each task condition and at each target location, as derived from the linear mixed model. These data show that the RT lags were more pronounced (a) after posterior than anterior AC TMS during the spatial task ( P <0.05, Tukey adjusted; N Subjects =10, N Trials/Subject =640) and (b) after anterior than posterior AC TMS during the identity task ( P <0.05, Tukey adjusted; N Subjects =10, N Trials/Subject =640). There was also a slightly weaker but significant main effect of TMS target location ( t =−2.2, P MCMC <0.05; N Subjects =10, N Trials/Subject =640). The main effect of task was non-significant, showing that there were no significant difficulty differences between the spatial and identity tasks. Group averages of RTs in different task conditions, separately for different TMS latencies, are shown in Table 1 . An additional analysis did not find any significant interactions between the task, target location and TMS pulse latency. Figure 2: TMS-induced RT lags during spatial and identity tasks. ( a ) Schematic illustration of the approximate TMS coil centre locations during bilateral anterior versus posterior stimulation. ( b ) Estimated marginal means and s.e. of RT lags derived from the linear mixed model, with the different stimulation latencies pooled together ( N =10). These data show a significant interaction between the task and TMS target factors, suggesting brain location-specific performance modulations during auditory identity versus spatial tasks. This result provides causal support for the theory of two distinct AC areas for sound identity and location processing [1] , [2] , which has previously been suggested in humans based on neuroimaging activation studies. * P <0.05, a priori comparison of task-specific effects across the TMS target loci derived from the linear mixed model; ††† P MCMC =0.001, task by target location interaction of the linear mixed model. Full size image Table 1 Group-average RTs in milliseconds. Full size table For hit rates (HRs), the linear mixed model did not indicate significant interaction effects between the task, target location and TMS treatment. TMS resulted in an overall decrease of 9% in HR (estimated marginal means±s.e. : 77±4% after TMS, 86±4% with no TMS; t 63 =4.1 , P <0.001; N Subjects =10, N Trials/Subject =640). The group estimates of HR values in the individual task conditions are shown in Table 2 . Finally, Fig. 3 shows the variability of task performance, quantified as the s.d. of RT, in each individual subject during the baseline trials, TMS trials and across all trials. Table 2 Group-average HR percentages. 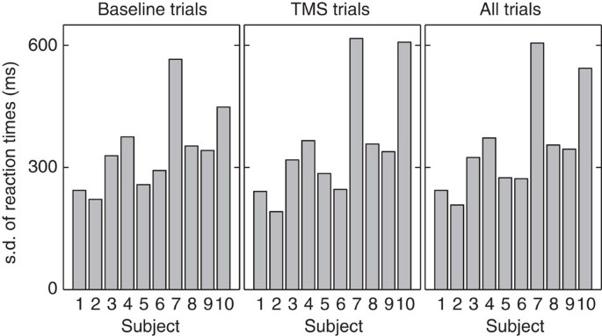Figure 3: The s.d. of individual-trial RTs in the population of 10 subjects. s.d. of RTs are shown during trials without TMS (left), during TMS (middle) and across all trials (right). The variance of RT performance was relatively homogeneous across subjects, apart from two subjects (7 and 10) who demonstrated a higher level of variance than the other subjects. This potential bias was taken into account in the linear mixed model by using least-squares weighting of the regression coefficients by the inverse variance of each subjects’ behavioural performance. Full size table Figure 3: The s.d. of individual-trial RTs in the population of 10 subjects. s.d. of RTs are shown during trials without TMS (left), during TMS (middle) and across all trials (right). The variance of RT performance was relatively homogeneous across subjects, apart from two subjects (7 and 10) who demonstrated a higher level of variance than the other subjects. This potential bias was taken into account in the linear mixed model by using least-squares weighting of the regression coefficients by the inverse variance of each subjects’ behavioural performance. Full size image Verifying TMS targeting by cortical E-field estimates The results of electromagnetic modelling analyses, which were conducted to verify the foci of E-fields induced by TMS in each subject, are shown in Fig. 4 . These data show that the intended targets were successfully stimulated during both posterior and anterior AC TMS conditions. The anterior AC stimulation reached maximal levels at areas anterolateral to Heschl’s gyrus, including anterior STG. The supratemporal areas stimulated during TMS of posterior AC included posterior STG and PT. Further, the E-field distributions were quite focal, resulting in that collateral fields (surrounding the intended target areas), which are largely unavoidable with TMS, did not extend to areas that have been associated with frontal or parietal auditory ‘what’ or ‘where’ pathways. For example, during the anterior TMS pulses, the supra-Sylvian fields reaching the threshold were centred at the central sulcus, far from IFG areas presumed to be associated with the auditory ‘what’ stream beyond AC. During posteriorly targeted TMS, the supra-Sylvian fields were strongest in inferior aspects of parietal cortex. The mean±s.d. distance along the supratemporal surface of peak E-field values between the anterior versus posterior stimulation sites was 34±10 mm ( N Subjects =10, N Pulse pairs/Location =160) in the left and 37±10 mm in the right hemisphere ( N Subjects =10, N Pulse pairs/Location =160). 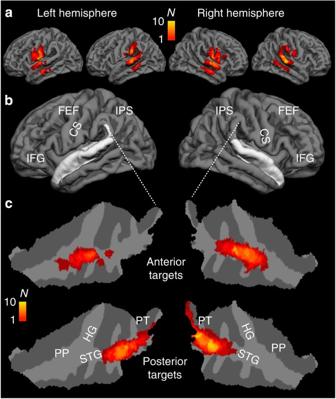Figure 4: Modeling of TMS-induced E-fields in the cortex. (a) Distribution of TMS effects exceeding 80% motor threshold strength during TMS in all subjects (N=10), shown on a standard brain cortical reconstruction. (b) Gross anatomical landmarks of interest shown on the standard brain cortex. The location of superior temporal cortices, which encompass ACs has been shown in white. The loci of central sulcus (CS), and extra-AC areas related to ‘what’ (inferior frontal gyrus, IFG) and ‘where’ (intraparietal sulcus, IPS; frontal eye fields, FEF) processing streams are also shown. (c) TMS-induced electric fields in AC on flattened patches of the superior temporal cortices. Taken together, our modelling results demonstrate that TMS-induced E-fields were successfully delivered at the posterior (posterior STG, PT) versus anterior AC areas (anterior STG, planum polare), hypothesized to be associated with sound location versus identity feature discrimination, respectively. As expected, TMS also induced E-fields in the adjacent cortical gyri. However, the panelashows that these fields were not close to the frontoparietal areas typically associated with extra-AC ‘where’ (IPS/FEF) and ‘what’ (IFG) processing. The colour scale depicts the number of subjects with stimulation reaching the threshold at a given location. Figure 4: Modeling of TMS-induced E-fields in the cortex. ( a ) Distribution of TMS effects exceeding 80% motor threshold strength during TMS in all subjects ( N =10), shown on a standard brain cortical reconstruction. ( b ) Gross anatomical landmarks of interest shown on the standard brain cortex. The location of superior temporal cortices, which encompass ACs has been shown in white. The loci of central sulcus (CS), and extra-AC areas related to ‘what’ (inferior frontal gyrus, IFG) and ‘where’ (intraparietal sulcus, IPS; frontal eye fields, FEF) processing streams are also shown. ( c ) TMS-induced electric fields in AC on flattened patches of the superior temporal cortices. Taken together, our modelling results demonstrate that TMS-induced E-fields were successfully delivered at the posterior (posterior STG, PT) versus anterior AC areas (anterior STG, planum polare), hypothesized to be associated with sound location versus identity feature discrimination, respectively. As expected, TMS also induced E-fields in the adjacent cortical gyri. However, the panel a shows that these fields were not close to the frontoparietal areas typically associated with extra-AC ‘where’ (IPS/FEF) and ‘what’ (IFG) processing. The colour scale depicts the number of subjects with stimulation reaching the threshold at a given location. Full size image Continuous tracking of the coils and head position with the navigation device indicated that movement was minimal during the experiment (group level mean of individually computed SDs for coil/head movements was 1.2 mm). This excludes the possibility that the differences between runs would have been caused by head/coil movements leading to stimulation of different brain areas. Here we studied the effects of transient focal AC deactivations induced by TMS [44] on processing of object identity versus spatial aspects of auditory stimuli. TMS pulse pairs targeted at anterior non-primary AC areas produced more pronounced RT lags during sound identity than location discrimination performance. In contrast, TMS targeted at posterior non-primary AC areas delayed RTs significantly more during the audiospatial than identity task. The linear mixed modelling analyses showed a corresponding significant interaction between the auditory task and anatomical target location on TMS-induced RT lags. These results provide direct causal support for distinct human AC regions for sound location and identity processing, which so far has been studied in healthy humans mainly using neuroimaging methods. The study also offers proof-of-principle for using TMS for studies on human AC functional anatomy. Previous studies have suggested that delivering ppTMS at the presently used intrapair interval of 2.5 ms triggers transient intracortical inhibition that lasts for up to a few tens of milliseconds [36] . Here the TMS pulses were delivered at four latencies between 55 and 145 ms after sound onset. This encompasses the time window during which the MEG/EEG response N1 typically ascends, peaks and descends in the posterior and anterior non-primary ACs (for example, refs 3 , 45 , 46 ). Notably, stimulus-locked neuronal processes occurring at these latencies at non-primary ACs are also believed to coincide with the emergence of conscious percepts and formation of neuronal representation of sound objects [45] , [46] . One might thus speculate that the present behavioural effects of TMS were caused by increased local inhibition that delayed sound-feature processing in the underlying areas. However, further studies are needed to verify the exact neuronal mechanisms of the presently observed effects. A large number of investigations in humans (for example, refs 1 , 2 , 3 , 11 , 12 , 13 , 14 ) and animal models [1] , [2] , [4] , even some of those supporting distributed coding instead of topographical representation of acoustic space [47] , [48] , are in line with the view that neurons processing spatial features are most abundantly populating the posterior auditory fields. As for the ‘what’ pathway, contradictory findings have been reported, for instance, in recent human neuroimaging studies that have found spread of pitch-related neuroimaging activations also to posterior AC [49] . This has been interpreted to contradict the existence of a pitch-specific region in the anterolateral AC, previously reported in monkeys [50] and humans (for example, refs 15 , 16 ). The present study, in which sound identity processing was measured using a task that required discrimination of AM differences (that is, temporal pitch), however, suggests that anterior AC areas may, indeed, be behaviourally relevant for pitch tasks. However, it is noteworthy that the present AM frequencies were slightly closer to the boundary of pitch versus flutter perception than the typical fundamental frequencies ( f 0 ) used in previous temporal-pitch functional MRI studies; for example, f 0 =62.5 Hz in ref. 51 and 83.1 Hz in ref. 15 . Thus, future studies may be needed to see how the present results generalize across different stimulus and task types. Although previous studies [3] , [45] , [46] have suggested a latency difference of about 10–30 ms between the N1 activation peaks in the posterior ‘where’ versus anterior ‘what’ regions, the present results regarding TMS latencies were inconclusive. That is, no significant interactions between the task type, TMS target and TMS latency emerged. Further studies could illuminate whether the interruption of local AC processes have characteristic critical latencies for different task types and subanatomical areas in humans. On the same note, the behavioural effects induced by TMS in the present study were, as fully expected because of the more transient nature of neuronal manipulations, more subtle than those produced by recent cooling deactivation studies [4] , which resulted in complete inactivation of larger extents of AC (and probably also in areas connected to the deactivated regions [28] , [29] ). Instead of a major decrease of HR, we observed RT delays <100 ms. Note also that the current extent of RT lags is logical, given the presumed short duration of neuronal effects of ppTMS. The present study demonstrates the utility of electromagnetic modelling of the TMS-induced E-fields at the individual cortical surfaces and the value of being able to compute surface-based across-subjects averages of the E-fields. To our knowledge, this is the first applied TMS study to report such data. Our modelling, specifically, showed that anterior and posterior TMS targeted separate areas in the intended regions, extending from the supratemporal cortex inside the Sylvian fissure to lateral aspects of STG that are more accessible to TMS than the core regions inside the sulcus. It is, however, noteworthy that beyond coil design and selection, TMS does not allow customized shaping of the E-fields, and volume conduction leads to that not only the maximum but also the immediately surrounding areas receive stimulation. For example, despite the fact that our study was based on an MRI-guided online navigation system and quite small stimulation coils that allow relatively focal targeting of cortical tissue, not only STG but also the adjacent gyri (albeit with lesser intensities) were stimulated. Yet, our electromagnetic modelling showed that, in the case of anterior AC stimulation, such ‘collateral’ TMS effects in supra-Sylvian regions were clearly more posterior than the inferior frontal ‘what’ stream (including the IFG areas pars opercularis and triangularis), as they actually peaked in the postcentral (that is, parietal lobe) regions. Similarly, in the case of the posterior AC target, the supra-Sylvian areas stimulated by ppTMS were restricted to the inferior aspects of parietal lobe and did not extend into the vicinity of the intraparietal sulcus, which is a key anatomical locus of the posterior parietal ‘where’ processing stream [1] , [52] . Most importantly, our estimates of TMS-induced E-fields showed clearest and most consistent foci across subjects in the anticipated AC areas. TMS coil discharges produce both auditory and somatosensory stimulations, which may cause auditory masking effects or nonspecific distractions on cognitive performance beyond the neuronal mechanisms of interest. For example, in the present study, ppTMS resulted also in nonspecific task modulations (RT increases to ppTMS, irrespective of target location) that might have been partially affected by these biases. (Note that, here, we used relatively small figure-of-eight of coils that produce less pronounced clicks than larger coils, as well as earpieces that dampen the click.) In previous studies, researchers have therefore applied several types of control conditions to separate the TMS effects of interest from artifacts. For example, one can apply either ‘sham TMS’ or real TMS to a control brain region that does not, presumably, participate in the activity of interest. A complication for using an independent ‘non-auditory’ control region is, however, that a wide network of areas beyond the supratemporal cortex is, either directly or through polymodal associations, activated during active auditory task performance. Indeed, auditory RTs have been shown to be affected by TMS delivered to a great variety of such ‘extra-auditory’ areas [38] , [39] , [40] , [41] . Therefore, in the present study, we applied a factorial design where each of the AC regions of interest, anterior versus posterior, acted as their own control during the two different auditory task domains. It is also noteworthy that the relatively high spatial focality and short (2.5-ms) duration of ppTMS would suggest that the behavioural effects emerge from local inhibition in the target area where SICI occurs. Although spreading influences to connected areas cannot be completely excluded, if present, they are probably much less prominent than those observed with deactivations lasting several orders of magnitude longer [30] , [31] , [32] , [33] , [34] used in animal models [4] . Finally, it is possible that certain extracerebral artifacts, such as scalp muscle stimulation, may result in feedback activities that might potentially cause more pronounced effects on processing of sound identity, particularly in the case of speech sounds [38] . Here such biases are probably less likely, as the present identity dimension was artificial, not directly linked to speech features. In summary, TMS to posterior AC regions delayed RTs significantly more during sound location than identity discrimination, whereas TMS to anterior AC regions delays RTs significantly more during sound identity than location discrimination. This double dissociation provides causal support for the parallel processing model [1] , [2] , [3] , [4] postulating that sound identity features are processed in anterior AC and sound location is encoded in posterior AC in humans. These results also demonstrate the potential usefulness of ppTMS for studying functional anatomy of the AC in humans, especially when combined with forward modelling of the TMS-induced E-fields on the cortical surface. Further studies are needed to verify the exact neuronal mechanisms that underlie the ppTMS cortical effects. Subjects and task design Ten healthy right-handed subjects (five women, age 22–51 years) with self-reported normal hearing, screened for TMS and MRI contraindications (metal in the body, implanted medical devices, medications affecting the central nervous system, pregnancy, history of seizures/convulsions/fainting/syncope or significant head trauma) [53] participated in the study. Human subjects’ approval was obtained and voluntary informed consents approved by the Massachusetts General Hospital Institutional Review Board were signed before the start of the experiment. TMS targeted at AC regions might stimulate temporal muscles, the intensity and discomfort of which varies across individuals. The subjects were informed that they could interrupt the experiment at any time, and their willingness to continue was confirmed repeatedly during the session. In each forced-choice RT trial ( Fig. 1a ), subjects were delivered a pair of binaural 300-ms white-noise bursts (50-dB sensation level, 10-ms on/off ramps) at a 1-s onset-to-onset interval (S14 Insert headphones, Sensimetrics, Malden, MA). The first sound of each pair was Reference, and the second was Probe. In the identity task, Probe was amplitude modulated (AM) at either one-sixth octaves lower (35.6 Hz) or higher (44.9 Hz) frequency than Reference (40-Hz AM frequency). After the lower-AM Probe, subjects were to press the leftmost of two buttons using their right-hand index finger, and after the higher-AM Probe the rightmost of these buttons with the right-hand middle finger. In the spatial task ( Fig. 1a ), References were simulated from 25° and Probes from either 20° or 30° to the right along the azimuth by convolving the Reference sound of the identity task (40 Hz AM) with generic head-related transfer functions [54] . The subjects were instructed to press the leftmost button with the right-hand index finger to the left Probes, and the rightmost button with the right-hand middle finger to the right Probes. Subjects received feedback in both tasks (‘OK’ or ‘Wrong’ shown during 0.9–1.9 s after each button press). The subsequent trial started 700 ms after the feedback stimulus ended. The trial duration (average across subjects 5.5 s) was, thus, paced by the subjects’ performance. The stimuli were presented and behavioural responses recorded on a PC running Presentation 14.2 (Neurobehavioral Systems, Albany, CA), which sent timing information to the TMS stimulators to synchronize the pulses with auditory stimuli. The difficulty of each task was matched a priori . Our statistical model (see below) showed no significant main effects of the task (identity versus spatial) for RTs or HRs, suggesting that the baseline difficulty levels of each task were consistent. ppTMS design TMS experiments were conducted in a dimly lit sound-attenuated low-reverberation chamber. The TMS coil navigation system was co-registered with each subject’s structural MRI (3T Siemens TimTrio, multi-echo MPRAGE pulse sequence, TR=2,510 ms; 4 echoes with TEs=1.64, 3.5, 5.36 and 7.22 ms; 176 sagittal slices, 1-mm isotropic voxels, 256 × 256 matrix; flip angle=7°) with respect to the fiduciary landmarks (nasion, two preauricular points) and additional scalp points using a 3D digitizer (Nexstim NBS, Helsinki, Finland). Two-channel TMS was guided with an infrared navigation system that calculates the location and strength of the induced E-field and displays this on the subject’s MRI in real time (Nexstim NBS). Subjects’ head movements were minimized by using a headrest and a vacuum pillow. During auditory stimulation/tasks, ppTMS (80/120% motor threshold of hand first dorsal interosseous; interpolated from previously reported optimal values [35] , [36] , [37] ) with 2.5-ms inter-pulse interval, biphasic waveform, was delivered simultaneously to both hemispheres with two stimulators (MagPro X100 w/MagOption, MagVenture, Falun, Denmark) and two figure-of-eight coils (MagPro C-B60, MagVenture). In separate runs, TMS was targeted either to anterior or posterior non-primary AC areas. TMS coil orientation was perpendicular to the individual local curvature of Sylvian fissure, (that is, about vertical). Bilateral TMS was chosen because sounds are processed simultaneously in both hemispheres, and because previous studies [4] suggest more consistent effects after bilateral than unilateral AC deactivations. Bilateral TMS, presumably, also helped avoid lateralized distraction effects during Spatial task. On the basis of previous studies [3] , [46] , the TMS pulse pairs were applied randomly at four different latencies (55, 85, 115 and 145 ms) after the Probe sound onset, covering the typical N1(m) activity in ACs. The experiment was divided into eight runs, each containing 80 trials and lasting on average 7 min 18 s. In each run, TMS was applied in 50% of trials in random order. Each session, thus, included 320 ppTMS events. On average, ppTMS was delivered about every 10–13 s. To avoid making the experiment excessively long, all conditions in one TMS location were always conducted in a row (coil re-targeting may require extra time when two coils are used). The order of TMS locations and task conditions was counterbalanced across subjects. Anatomical ppTMS target definition Each subject’s anatomical MRIs were segmented and co-registered to volume-based and surface-based standard brain representations using FreeSurfer 5.1 ( http://www.surfer.nmr.mgh.harvard.edu ). The TMS target locations were selected based on a sample of previously published maximally activated functional MRI [10] , [11] , [13] , [14] , [15] , [16] and positron emission tomography [51] voxels during audiospatial or sound-object identity processing. More specifically, the posterior AC targets were defined by averaging the peak-voxel Talairach coordinates of contrasts reflecting sound movement versus rest [11] , sound direction changes versus constant stimulation [13] , sound distance versus intensity changes [14] and spatially shifting versus stationary sounds [10] . When needed, Montreal Neurological Institute coordinates were converted to Talairach coordinates. The anterior AC targets were defined similarly, based on peak voxels in contrasts reflecting varying versus fixed pitch [10] , [15] , [16] , fixed pitch versus noise [15] , fixed Huggins pitch versus noise [16] , fixed binaural band pitch versus noise [16] and pitch-strength-by-melody interactions [51] . For both targets, average loci were calculated first within, and then across studies. The resulting Talairach coordinates (mm) of initial targets were { x,y,z }={−52,−30,12} for the left posterior, { x,y,z }={−54,0,−5} for the left anterior, { x,y,z }={60,−30,11} for the right posterior and { x,y,z }={55,−4,−6} for the right anterior AC ( Fig. 1b ). These locations were then transformed to each individual subject’s brain representations. Finally, before the TMS experiment, an optimized entry point closer to the inner skull was selected, as guided by the E-field estimates produced by the navigation system, to allow the TMS effects to be maximally focused to the target area. TMS target post hoc confirmation Electromagnetic modelling analyses utilizing realistic anatomy were conducted to estimate the actual cortically induced E-field distributions in each subject. The inner skull surface obtained from Freesurfer MRI reconstructions was used to create a single-layer boundary element model. The intracranial space was considered as a homogenous isotropic volume conductor. The position and orientation of the TMS coil was exported from the navigator computer in the MRI coordinates and a model for the wire winding geometry was constructed according to the manufacturer’s specifications (MagPro C-B60, MagVenture). TMS-induced E-field amplitudes were computed at the white matter surfaces (extracted using Freesurfer) according to the well-established physical principles, as described by Nummenmaa et al . [55] . The custom implementation of the numerical methods was done in Matlab (R2012a, The Mathworks, Inc., Natick, MA) utilizing the core routines from the boundary element model toolbox of ref. 56 . For comparisons across subjects, the cortical activation estimates were co-registered via spherical morphing to a surface-based standard brain representation [57] , thresholded at 80% of the individual’s maximum and normalized across individuals. Data analysis A full factorial design was utilized to control for potential biases caused by the TMS side effects (acoustic clicks and muscle stimulation). Behavioural data, including RTs (correct responses only) and HRs, were recorded separately for each task condition. At the initial screening, trial responses faster or slower than two s.d. of each subject’s average RT were excluded as outliers (physiologically unreasonable responses, that is, RT<50 ms or >4 s, were excluded before this). Statistical analyses were conducted using the R packages lme4, languageR and lsmeans [58] , [59] , [60] . Instead of averaging RTs first within subjects, we utilized a linear mixed approach [42] , [43] that models individual responses in each task condition/subject and brings the potential longitudinal biases between successive trials into the statistical model specification. To further mitigate within-session fluctuations (for example, related to the blocked TMS design), we specifically examined the time series of TMS-induced RT lags obtained by subtracting the within-condition average RT Baseline from each individual RT TMS event. The RT lag time series were finally entered into a linear mixed model: The random effects included the subject and trial type (sound direction nested within spatial task; AM frequency nested within identity task); the fixed effects included the task (identity versus spatial), TMS target location (anterior versus posterior), task-by-TMS-target–location interaction, TMS pulse-pair latency (55–145 ms), age, gender and the trial-specific sequential predictors (task-block number, trial numbers and RT to preceding baseline trial) controlling for temporal dependencies/autocorrelations. We controlled for potential biases caused by non-normality and homogeneity by examining the model residuals against fitted values. Multicollinearity was addressed by residualizing predictors correlating with each other. The model was weighted by the inverse variances of each subject’s behavioural performance. Our main hypothesis regarded the interaction between the task and TMS target location: we hypothesized that RT lags are significantly larger with TMS targeted to the anterior versus posterior AC during the identity task, and vice versa during the spatial task. Statistical significances were presented as MCMC-estimated P -values. A priori comparisons were computed based on the main models using the R lsmeans package [60] . Finally, HR results were analysed with a linear mixed model with the task, target location, treatment (TMS versus no TMS), age and gender as fixed-effect factors and the subject as a random-effect factor. How to cite this article: Ahveninen, J. et al . Evidence for distinct human auditory cortex regions for sound location versus identity processing. Nat. Commun. 4:2585 doi: 10.1038/ncomms3585 (2013).